Surface transfer doping induced effective modulation on ambipolar characteristics of few-layer black phosphorus Black phosphorus, a fast emerging two-dimensional material, has been configured as field effect transistors, showing a hole-transport-dominated ambipolar characteristic. Here we report an effective modulation on ambipolar characteristics of few-layer black phosphorus transistors through in situ surface functionalization with caesium carbonate (Cs 2 CO 3 ) and molybdenum trioxide (MoO 3 ), respectively. Cs 2 CO 3 is found to strongly electron dope black phosphorus. The electron mobility of black phosphorus is significantly enhanced to ~27 cm 2 V −1 s −1 after 10 nm Cs 2 CO 3 modification, indicating a greatly improved electron-transport behaviour. In contrast, MoO 3 decoration demonstrates a giant hole-doping effect. In situ photoelectron spectroscopy characterization reveals significant surface charge transfer occurring at the dopants/black phosphorus interfaces. Moreover, the surface-doped black phosphorus devices exhibit a largely enhanced photodetection behaviour. Our findings coupled with the tunable nature of the surface transfer doping scheme ensure black phosphorus as a promising candidate for further complementary logic electronics. Two-dimensional (2D) layered materials such as graphene and transition metal dichalcogenides (TMDs) have been considered as promising building blocks for the next-generation nanoelectronic devices, showing great potentials to extend the scaling limits existing in silicon-based complementary metal oxide semiconductor field effect transistors (CMOS-FET) [1] , [2] , [3] , as well as to serve as a high-mobility alternative to organic semiconductors for flexible electronic and optoelectronic devices [4] , [5] . Graphene, as the forefather of 2D materials [6] , has exhibited extremely high carrier mobility (>100,000 cm 2 V −1 s −1 ; ref. 7 ) and a wealth of fundamental physical properties [8] , [9] , [10] . However, graphene-based electronic devices seriously suffer from the absence of an intrinsic bandgap, which strongly limits the application of graphene in logic electronics [11] . Recently, TMDs with an inherent bandgap have emerged as promising materials for both electronic and optoelectronic applications [12] , [13] , [14] . Among the TMD family, molybdenum disulfide (MoS 2 ) FET devices mostly present the n-type semiconducting behaviour attributed to the intrinsic atomic defects of MoS 2 , such as sulfur vacancies, as well as the pronounced Fermi level pinning effect at metal contacts/MoS 2 interface [15] , [16] , which severely restricts its applications in both CMOS transistors and p–n diodes [17] , [18] . Tungsten diselenide (WSe 2 ), another member in 2D TMDs, demonstrates the great possibility to be fabricated as complementary logic devices on a single flake resulting from its ambipolar transport characteristics [19] , [20] , [21] . Nevertheless, the device performance of WSe 2 FETs strongly depends on the metal contacts, showing limited carrier mobility without sufficient contact doping [13] , [22] . Therefore, to further develop atomically thin 2D semiconductors based CMOS electronics, the newly discovered p-type or ambipolar 2D materials with high carrier mobility are highly desirable. Black phosphorus (BP), a fast emerging 2D material, was recently isolated from the layered BP crystals, where each phosphorus atom is covalently bonded to three neighbouring atoms to form the puckered orthorhombic structure [23] , [24] . BP has a direct bandgap for all number of layers, predicted from 0.3 eV for bulk to 2 eV for monolayer [25] , [26] , [27] , [28] . This characteristic leads to remarkable applications for BP-based optoelectronic devices [24] , [29] . Moreover, the intrinsic small bandgap allows the few-layer BP to be easily modulated between ON and OFF conduction states. The multilayer BP-configured FET devices demonstrate the clear ambipolar transport behaviour with remarkably high hole mobility up to ~1,000 cm 2 V −1 s −1 and on/off ratio of ~10 5 at room temperature [23] , [30] , making this material suitable for transistors. On the other hand, the ambipolar characteristics of BP FETs show the strong asymmetry between electron and hole transport [31] , where both the concentration and mobility of electrons are orders of magnitude lower than that of holes, making it difficult to fulfil the complementary logic devices on a single BP flake. In order to better control and further enhance the performance of BP-based complementary devices, it is of great significance to effectively tune the n- or p-type doping level of BP. Chemical doping, as a simple and effective doping approach, has been widely utilized to manipulate the electronic properties of 2D materials as well as organic semiconductors [13] , [32] , [33] , [34] , [35] , [36] . Compared with the electrostatic modulation via an external electrical field, chemical doping usually provides a stronger non-volatile doping capability with the ease of device fabrication [37] . Surface transfer doping relies on the interfacial charge transfer without introducing significant defects into the lattice structure of the as-doped materials, thereby nearly reserving their fundamental transport properties [38] . Various organic and inorganic species have demonstrated excellent doping effects on 2D materials such as graphene and TMDs, among which caesium carbonate (Cs 2 CO 3 ) and molybdenum trioxide (MoO 3 ) have been used to effectively modify the doping level of MoS 2 and grapheme, respectively [32] , [33] . Furthermore, the contact doping on TMDs FETs, such as MoS 2 and WSe 2 , has been shown to remarkably enhance the device performance owing to the effective modulation of Schottky barrier formed at contact/semiconductor interface [13] , [36] . In the following, we report the surface transfer electron and hole doping to effectively tune the ambipolar characteristics of few-layer BP FETs via in situ surface functionalization with Cs 2 CO 3 and MoO 3 . The BP device is found to be strongly n-type doped by Cs 2 CO 3 layer. The electron mobility of BP is significantly increased to ~27 cm 2 V −1 s −1 after 10 nm Cs 2 CO 3 decoration, which leads to highly improved electron transport in BP devices. On the other hand, MoO 3 shows a marked p-type doping effect on BP devices with non-degraded hole mobility. In situ ultraviolet photoelectron spectroscopy (UPS) and X-ray photoelectron spectroscopy (XPS) characterization confirm the interfacial charge transfer between BP and doping layers. This doping can also modulate the Schottky junctions formed between metal contacts and BP flakes, and hence to enhance the photoresponsivity of BP-based photodetectors. 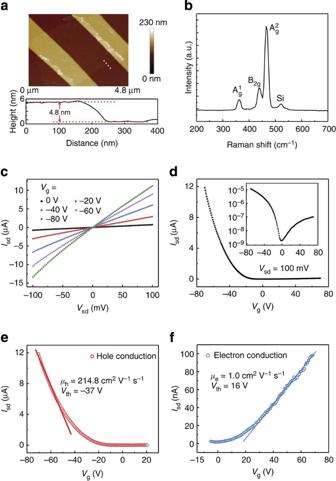Figure 1: Few-layer back-gated BP field effect transistor and device characterization. (a) Atomic force microscopy image of an as-fabricated BP device. The line profile at the edge of the BP flake indicates a multilayer BP crystal of ~4.8 nm (~8 layers). (b) RAMAN spectroscopy of BP flake used for device fabrication. (c)Isd–Vsdcharacteristics of a BP FET as a function of different gate voltages from 0 to −80 V. (d) Transfer characteristics (Isd–Vg) of the same device withVsd=100 mV. Inset: logarithmic plot of the transfer curve. Separate transfer curves for (e) hole and (f) electron conduction, respectively;μhandμeare the hole and electron mobility respectively;Vthis the threshold voltage. Characterization of BP FET devices Figure 1a displays the atomic force microscopy image of an as-made BP FET device on highly p-doped silicon substrate with 300 nm SiO 2 . The line profile reveals the BP flake thickness of ~4.8 nm, that is, ~8 atomic layers. As illustrated in Fig. 1b , the first-order Raman spectrum of exfoliated few-layers BP exhibits the characteristic peaks nearly located at 364, 438 and 465 cm −1 , corresponding to the three different vibration modes A 1 g , B 2g and A 2 g in BP crystal lattice, respectively [39] . Figure 1: Few-layer back-gated BP field effect transistor and device characterization. ( a ) Atomic force microscopy image of an as-fabricated BP device. The line profile at the edge of the BP flake indicates a multilayer BP crystal of ~4.8 nm (~8 layers). ( b ) RAMAN spectroscopy of BP flake used for device fabrication. ( c ) I sd –V sd characteristics of a BP FET as a function of different gate voltages from 0 to −80 V. ( d ) Transfer characteristics ( I sd –V g ) of the same device with V sd =100 mV. Inset: logarithmic plot of the transfer curve. Separate transfer curves for ( e ) hole and ( f ) electron conduction, respectively; μ h and μ e are the hole and electron mobility respectively; V th is the threshold voltage. Full size image Figure 1c exhibits the typical source-drain current versus source-drain voltage ( I sd –V sd ) characteristics of the fabricated BP FETs under different gate voltages measured under high vacuum (10 −8 mbar). Excellent linearity with V sd ranging from −100 to 100 mV suggests the good contact between the metal electrodes and the BP flake. The transfer characteristic ( I sd –V g ) of the same device is shown in Fig. 1d . Applying the gate voltage ranging from −70 to 70 V, the source-drain current under 100 mV bias increased along both negative and positive sweeping directions, corresponding to the hole and electron transport, respectively. This indicates a typical ambipolar transport behaviour. Moreover, a much faster current increase was observed in the negative gate voltage region compared with that of the positive side, revealing a hole-transport-dominated ambipolar characteristic. The inset logarithmic plot shows the I on / I off ratio of this BP-based FET to be ~10 4 , which is in good agreement with the previously reported values [23] , [30] . The threshold voltage V th of the ambipolar device was determined to be approximately −37 V for holes and ~16 V for electrons, extracted from the linear extrapolation of current onset in the linear region of hole and electron side, respectively ( Fig. 1e,f ). Based on the transfer plot, the carrier concentration induced by gate voltage V g in the linear region was estimated by the formula below: where C i is the capacitance per unit area between BP and back gate given by C i = ε 0 ε r / d , and ε r , d are the dielectric constant and thickness of SiO 2 , respectively. For example, the hole concentration at V g =−50 V was derived to be 9.3 × 10 11 cm −2 ; while the electron concentration can be estimated to be 1.0 × 10 12 cm −2 under V g =40 V. Similarly, the field effect carrier mobility of BP flake can be evaluated via the equation: where d I sd /d V g represents the maximum slope extracted from the linear region of transfer characteristic, L and W are the length and width of conduction channel, respectively. For the device illustrated in Fig. 1d , the hole and electron mobility were calculated to be 214.8 and 1.0 cm 2 V −1 s −1 , respectively. Surface transfer electron doping on BP devices by Cs 2 CO 3 Cs 2 CO 3 , as an efficient electron-donating material, has been extensively utilized in organic electronics owing to its low work function [40] , [41] . In order to explore the surface functionalization of Cs 2 CO 3 on tuning the electrical transport properties of BP, Cs 2 CO 3 was in situ evaporated onto the fabricated devices in high vacuum. 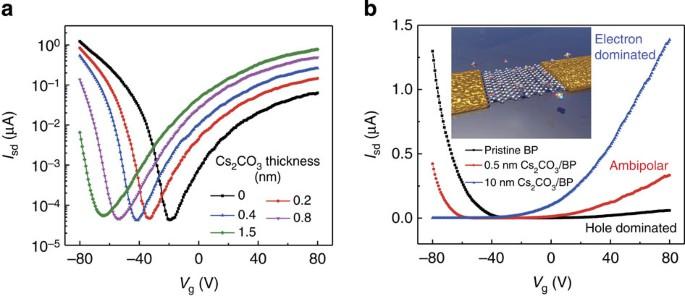Figure 2: Transfer characteristics evolution for Cs2CO3-modified BP field effect transistor. (a) Forward transfer characteristics (Vgfrom −80 to 80 V) evolution of a BP FET measured atVsd=100 mV in logarithmic scale with increasing Cs2CO3thickness from 0 to 1.5 nm. (b) Linear plot of the transfer curves at 0.5 and 10 nm Cs2CO3coverage with respect to the pristine BP. The electron transport of BP FET was significantly improved after Cs2CO3modification, leading to either a more balanced ambipolar or even electron-transport-dominated FET characteristic. Inset: schematic illustration of BP device coated by Cs2CO3. Figure 2a demonstrates the typical forward transfer characteristics evolution ( V g from −80 to 80 V) in logarithmic scale of BP devices with increasing Cs 2 CO 3 thickness. The initial transfer curve without Cs 2 CO 3 presents a current minimum of approximately −19 V. As the thickness of Cs 2 CO 3 increased to 1.5 nm, the current minimum progressively moved to ~−64 V. This suggests a significant n-type doping effect on Cs 2 CO 3 -decorated BP, originating from the interfacial electron transfer from Cs 2 CO 3 to BP owing to the large work function difference between them. The backward gate sweeping ( V g from 80 to −80 V) was also implemented on the same Cs 2 CO 3 -doped BP device ( Supplementary Fig. 1 ). The transfer curve presents the similar negative shifting with increasing Cs 2 CO 3 thickness. This indicates that such strong n-type doping effect of Cs 2 CO 3 on BP applies to both forward and backward gate sweeping in spite of large hysteresis in BP FETs, as discussed in Supplementary Note 1 . The transfer curves coated by 0.5 and 10 nm Cs 2 CO 3 were plotted with respect to pristine BP in linear scale as shown in Fig. 2b . At 0.5 nm Cs 2 CO 3 coverage, the on-current in electron regime almost reached the same level as that of the hole regime, demonstrating a more symmetric and balanced ambipolar characteristic. With even higher Cs 2 CO 3 coverage, the current of electron side gradually evolved beyond the hole side, which indicates an electron-transport-dominated ambipolar behaviour. After 10 nm Cs 2 CO 3 deposition, pure n-type transport characteristic was reached in the limited gate voltage range for the modified BP device. The calculated electron concentration ( V g =30 V) and mobility were plotted as a function of Cs 2 CO 3 thickness in Fig. 3a . The estimated electron concentration of BP at 30 V V g clearly increased from 5.0 × 10 11 to 1.5 × 10 12 cm −2 with the gradual deposition of Cs 2 CO 3 . More intriguingly, the Cs 2 CO 3 -functionalized BP device presents almost 25 times enhancement of electron mobility from 1.1 cm 2 V −1 s −1 for pristine BP to 27.1 cm 2 V −1 s −1 at 10 nm Cs 2 CO 3 coverage, revealing a remarkably improved electron transport in the BP channel. We propose that the undoped BP possesses high concentration of charge (electron) trapping sites, and hence the low electron mobility of undoped BP is mainly limited by the trapped charge scattering. The n-type doping can largely increase electron concentration to fill these trapping sites as well as to effectively screen the trapped charges, and hence the electron mobility can greatly increase as shown in Fig. 3a . Alternatively, the electron doping in BP can also reduce the effective Schottky barrier height between BP and metal contacts, which makes the electron transport in BP not limited by contacts and approach to its intrinsic transport behaviours. In order to figure out the contact resistance between metal electrodes and doped BP channel, four-terminal measurements were also performed on Cs 2 CO 3 -modified BP devices. As illustrated in Supplementary Fig. 2 , the transfer characteristics measured by four-terminal configuration did not show much difference from two-terminal configuration for all Cs 2 CO 3 thickness, resulting from the much lower contact resistance compared with the channel resistance ( Supplementary Table 1 ). Moreover, the extracted contact resistance largely decreased with increasing Cs 2 CO 3 thickness as predicted, which will be discussed in the last part. This reveals that the contacts between metal and BP channel do not clearly restrict the BP FET performance, and thus the performance enhancement of Cs 2 CO 3 -decorated BP devices (for example, electron mobility enhancement) mainly originates from the improved intrinsic transport properties of BP channel, not reduced contact resistance ( Supplementary Note 2 ). Owing to the remarkably enhanced electron mobility and concentration, the conductivity of BP was largely increased from 0.01 to 1.37 μS by two orders of magnitudes after 10 nm Cs 2 CO 3 deposition, as presented in Fig. 3b . Although the undoped multilayer BP FETs could operate in either hole or electron-transport regime, both the source-drain current and mobility in the electron side are much lower than that of the hole side at equal back gate doping levels. Our results demonstrate that Cs 2 CO 3 overlayers can serve as an efficient n-type surface dopant to effectively improve the electron transport in BP devices, thereby inducing either a more balanced ambipolar or even electron-transport-dominated FET behaviour. Figure 2: Transfer characteristics evolution for Cs 2 CO 3 -modified BP field effect transistor. ( a ) Forward transfer characteristics ( V g from −80 to 80 V) evolution of a BP FET measured at V sd =100 mV in logarithmic scale with increasing Cs 2 CO 3 thickness from 0 to 1.5 nm. ( b ) Linear plot of the transfer curves at 0.5 and 10 nm Cs 2 CO 3 coverage with respect to the pristine BP. The electron transport of BP FET was significantly improved after Cs 2 CO 3 modification, leading to either a more balanced ambipolar or even electron-transport-dominated FET characteristic. Inset: schematic illustration of BP device coated by Cs 2 CO 3 . 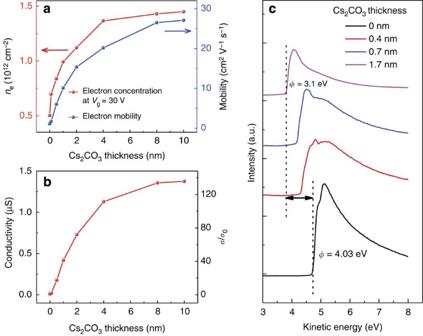Figure 3: Analysis of electrical transport properties and UPS evolution for Cs2CO3-coated BP. (a) Electron concentration (ne) atVg=30 V and mobility of BP versus Cs2CO3thickness. The electron mobility is remarkably enhanced by ~25 times to ~27 cm2V−1s−1. (b) The plot of BP conductivity (σ) at zero gate voltage as a function of electron concentration.σ0is the conductivity of pristine BP. (c) UPS spectra evolution at the low kinetic energy region (secondary electron cutoff) with respect to the Cs2CO3thickness.Φis the work function. Full size image Figure 3: Analysis of electrical transport properties and UPS evolution for Cs 2 CO 3 -coated BP. ( a ) Electron concentration ( n e ) at V g =30 V and mobility of BP versus Cs 2 CO 3 thickness. The electron mobility is remarkably enhanced by ~25 times to ~27 cm 2 V −1 s −1 . ( b ) The plot of BP conductivity ( σ ) at zero gate voltage as a function of electron concentration. σ 0 is the conductivity of pristine BP. ( c ) UPS spectra evolution at the low kinetic energy region (secondary electron cutoff) with respect to the Cs 2 CO 3 thickness. Φ is the work function. Full size image In situ UPS/XPS measurements were carried out on Cs 2 CO 3 -coated bulk BP to further understand the interfacial interaction between Cs 2 CO 3 and BP. The evolution of the UPS spectra at the low kinetic energy region with respect to Cs 2 CO 3 thickness is exhibited in Fig. 3c . By linearly extrapolating the low kinetic energy onset in UPS spectra, the work function of natural bulk BP was measured to be 4.03 eV. After 1.7 nm Cs 2 CO 3 deposition, the work function sharply decreased to 3.1 eV, originating from the substantial interfacial electron transfer from Cs 2 CO 3 to BP. This significant charge transfer was also confirmed by the XPS core level spectra of P 2p 3/2 , as shown in Supplementary Fig. 3 . With increasing Cs 2 CO 3 thickness, the P 2p 3/2 peak gradually shifted to higher binding energy region. This indicates a downward band bending of ~0.2 eV coated by 1.7 nm Cs 2 CO 3 , originating from the increase of electron concentration in Cs 2 CO 3 -doped BP, and therefore the Fermi level of BP moving closer to the conduction band edge. Surface transfer hole doping on BP devices by MoO 3 In contrast to the electron doping via Cs 2 CO 3 , thermally grown MoO 3 layers in high vacuum possess the extremely high work function of ~6.8 eV (ref. 42 ), and thereby create giant hole-doping effect on few-layer BP FETs. As presented in Fig. 4a , the pristine BP FET exhibits the current minimum located at ~21 V. When the MoO 3 thickness increased to 0.1 nm, the current minimum positively shifted to ~67 V, indicating a marked p-type doping effect of MoO 3 on BP device. Moreover, the transfer curve kept positively shifting with even higher MoO 3 thickness, where the threshold voltage was unreachable for the limited safe gate voltage compliance. It is worth noting that MoO 3 exhibited similar p-type doping effects on BP in bidirectional gate sweeping ( Supplementary Fig. 4 ), suggesting that the existing hysteresis in BP device does not affect the doping effect of MoO 3 . Similar to the Cs 2 CO 3 doping case, the hole concentration ( V g =−30 V) and mobility was extracted and plotted with respect to MoO 3 thickness in Fig. 4b . After depositing 12 nm MoO 3 , the hole concentration of BP at −30 V V g was increased from 1.6 × 10 12 to 5.8 × 10 12 cm −2 ; while the hole mobility almost remained unchanged at ~200 cm 2 V −1 s −1 even at the high doping level covered by over 10 nm MoO 3 . Such retained hole mobility reveals that the hole transport in MoO 3 -doped BP was dominated by phonon scattering, and the charge–charge scattering can be ignored in spite of the strongly enhanced hole concentration after doping. After 12 nm MoO 3 decoration, the conductivity of BP FET was largely enhanced from 1.6 to 57.9 μS (inset of Fig. 4b ). Four-terminal characterizations on MoO 3 -modified BP devices ( Supplementary Fig. 5 and Supplementary Table 2 ) further exhibit much lower contact resistance compared with the channel resistance during MoO 3 deposition. 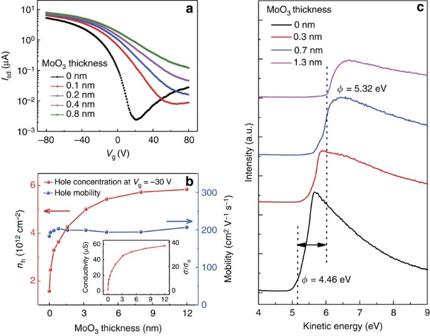Figure 4: Hole doping of BP field effect transistor via MoO3modification. (a) Forward transfer characteristics (Vgfrom −80 to 80 V) evolution of a separate BP FET measured atVsd=100 mV with respect to the MoO3thickness from 0 to 0.8 nm. (b) Hole concentration (nh) atVg=−30 V and mobility of BP versus MoO3thickness. Inset: BP conductivity at zero gate voltage as a function of MoO3thickness. (c) UPS spectra evolution at lower kinetic energy region with increasing MoO3coverage. Figure 4: Hole doping of BP field effect transistor via MoO 3 modification. ( a ) Forward transfer characteristics ( V g from −80 to 80 V) evolution of a separate BP FET measured at V sd =100 mV with respect to the MoO 3 thickness from 0 to 0.8 nm. ( b ) Hole concentration ( n h ) at V g =−30 V and mobility of BP versus MoO 3 thickness. Inset: BP conductivity at zero gate voltage as a function of MoO 3 thickness. ( c ) UPS spectra evolution at lower kinetic energy region with increasing MoO 3 coverage. Full size image Similarly, in situ UPS/XPS measurements on MoO 3 covered bulk BP were also conducted to examine the underlying interfacial charge transfer mechanism between MoO 3 and BP. As exhibited in Fig. 4c , the UPS spectra of bulk BP gradually evolved towards the higher kinetic energy region with increasing MoO 3 thickness, suggesting that the strong work function increase from 4.46 to 5.32 eV after the deposition of 1.3 nm MoO 3 . Owing to the high work function of MoO 3 , significant electron transfer from BP to MoO 3 occurred at the MoO 3 /BP interface. Furthermore, the obvious upward bend banding was observed in P 2p 3/2 core level XPS spectra with MoO 3 deposition, as shown in Supplementary Fig. 6 , indicating the increase of hole concentration in MoO 3 -doped BP. Photodection behaviour of chemically doped BP devices Arising from a predicted direct bandgap for all number of layers, BP has been used for ultrafast and wide spectrum response photodetectors [29] . In this work, we also evaluated the photodetection properties of BP FETs doped by MoO 3 and Cs 2 CO 3 layers. The in situ photoresponse measurements were performed by the illumination of a 405-nm laser with the light power of 40 mW (spot diameter 2 mm) exactly after the deposition of surface doping layers in high vacuum chamber. 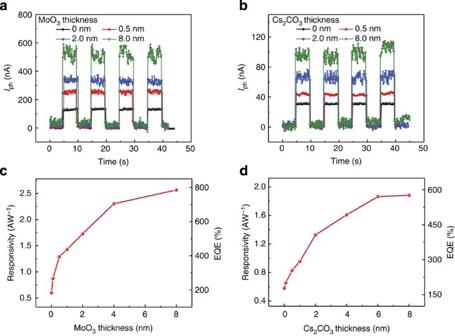Figure 5: Time-dependent photoresponse for surface transfer-doped BP photodetectors. Time dependence of photocurrent measured atVsd=3 V upon the illumination of a 405-nm laser source with the power of 40 mW (spot diameter 2 mm) with thein situdeposition of (a) MoO3and (b) Cs2CO3. Calculated photoresponsivity and EQE as a function of (c) MoO3and (d) Cs2CO3thickness. Figure 5a,b shows the time-dependent photoresponse characteristics of BP photodetector with the gradually increased MoO 3 and Cs 2 CO 3 thickness, respectively, at V sd =3 V and V g =0 V. The apparent photocurrent enhancement was both identified with increasing MoO 3 and Cs 2 CO 3 thickness. After 8.0 nm deposition, the excited photocurrent was largely increased by 3–4 times for both MoO 3 and Cs 2 CO 3 cases. Furthermore, the doping process did not severely degrade the response time of BP photodetector, as illustrated in Supplementary Figs 7 and 8 , where the rising and decaying time nearly remained at several milliseconds level with increased dopant coverage. Figure 5: Time-dependent photoresponse for surface transfer-doped BP photodetectors. Time dependence of photocurrent measured at V sd =3 V upon the illumination of a 405-nm laser source with the power of 40 mW (spot diameter 2 mm) with the in situ deposition of ( a ) MoO 3 and ( b ) Cs 2 CO 3 . Calculated photoresponsivity and EQE as a function of ( c ) MoO 3 and ( d ) Cs 2 CO 3 thickness. Full size image The photoresponsivity ( R ) and external quantum efficiency (EQE), as two critical parameters of photodetector performance, were calculated and plotted as a function of dopant thickness in Fig. 5c,d . R is defined as the photocurrent generated by per unit power of incident light on the effective area of a photodetector; while EQE is the number of carriers circulating a photodetector per absorbed photon and per unit time [43] ; where I ph is the photocurrent induced by incident light, S is the effective area under illumination, P is the light intensity and λ is the wavelength of incident light, and h , c and e represent the Plank constant, velocity of light and the charge of electron, respectively. After depositing 8.0 nm doping layers, the responsivity of MoO 3 -decorated BP photodetector increased from 0.6 to 2.56 AW −1 ; while Cs 2 CO 3 modification improved the responsivity from 0.58 to 1.88 AW −1 . This surface transfer doping enhanced responsivity is much higher than the previously reported BP photodetector [29] , even higher than some reported TMDs-based photodetectors, such as MoS 2 (refs 14 , 44 ) and WS 2 (ref. 45 ). Moreover, the MoO 3 and Cs 2 CO 3 decoration improved the corresponding EQE from 183% to 784% and from 178% to 576%, respectively, demonstrating an excellent performance enhancement for surface-functionalized BP photodetectors. The mechanism of the surface doping enhanced photoresponse for BP photodetector is proposed by the modulation of Schottky junction formed at the metal contacts/BP interface, as shown in Fig. 6 . Before the application of source-drain bias, the energy level alignment between metal electrodes and BP reached the equilibrium once the physical contacts were established, indicating a non-negligible Schottky barrier between metal contact and BP flake. Upon the illumination of BP device with a source-drain bias, the photo-generated charge carriers in BP channel could undergo a thermal-assisted tunnelling process passing through the Schottky barrier to metal electrode, which contributes to the increase of channel current ( Fig. 6b ). After the effective hole doping on BP channel by MoO 3 , as shown in Fig. 6c , the Fermi level was dragged downwards to the valence band of BP, which compress the Schottky barrier region, and thus reduce the effective barrier height as well as the contact resistance. This significantly facilitates the electrical transport of photo-induced holes, thereby leading to the apparent photocurrent enhancement. Similarly, the electron doping of Cs 2 CO 3 pulled the Fermi level towards the BP conduction band, which narrows the Schottky barrier and lowers the contact resistance for electron transport in BP channel. Therefore, the photo-induced electrons could penetrate the barrier more easily, producing the enhanced photoresponse for Cs 2 CO 3 -modified devices. 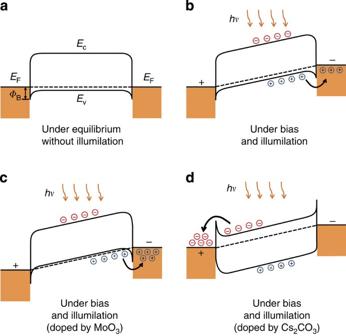Figure 6: Qualitative energy band diagrams of BP device through surface transfer doping. Energy band structures between metal contacts and BP (a) without and (b) with source-drain bias for pristine BP. Energy level alignment with source-drain bias after (c) MoO3and (d) Cs2CO3doping.EFis the Fermi level energy.ΦBis the Schottky barrier height.ECandEVrepresent the minimum energy of conduction band and the maximum energy of valance band, respectively. The Schottky barrier formed at metal/BP interface was compressed for both hole and electron doped BP device, facilitating the tunnelling transport of photon excited charge carriers. All the experiments were replicated at least 10 times on separate devices. Figure 6: Qualitative energy band diagrams of BP device through surface transfer doping. Energy band structures between metal contacts and BP ( a ) without and ( b ) with source-drain bias for pristine BP. Energy level alignment with source-drain bias after ( c ) MoO 3 and ( d ) Cs 2 CO 3 doping. E F is the Fermi level energy. Φ B is the Schottky barrier height. E C and E V represent the minimum energy of conduction band and the maximum energy of valance band, respectively. The Schottky barrier formed at metal/BP interface was compressed for both hole and electron doped BP device, facilitating the tunnelling transport of photon excited charge carriers. All the experiments were replicated at least 10 times on separate devices. Full size image In this article, we demonstrate effective surface transfer electron and hole doping on few-layer BP FET devices through in situ surface functionalization with Cs 2 CO 3 and MoO 3 overlayers, respectively. The electron mobility of BP FETs is found to be significantly enhanced to ~27 cm 2 V −1 s −1 after 10 nm Cs 2 CO 3 modification, giving rise to a highly improved electron transport in the ambipolar characteristics of BP. In contrast, MoO 3 exhibits giant hole-doping effects on BP devices accompanied by the nearly maintained hole mobility of ~200 cm 2 V −1 s −1 . The photodetecting behaviours of surface-doped BP devices are also carefully probed. The responsivity of BP photodetectors is largely enhanced to 2.56 and 1.88 AW −1 without degrading response speed after 8.0 nm MoO 3 and Cs 2 CO 3 doping, respectively. Our results promise a simple method to either electron or hole dope BP, and thus effectively tailor the ambipolar characteristics of BP FETs to realize the high-performance BP-based complementary logic circuit as well as other functional electronic and optoelectronic devices. Sample preparation and device fabrication Few-layer BP flakes were mechanically exfoliated from bulk BP crystals (Smart Elements) using a scotch tape and transferred onto degenerately p-type-doped silicon wafers coated with 300 nm SiO 2 . Exactly after locating the exfoliated BP flake by using high-resolution microscope (Nikon Eclipse LV100D), photoresist PMMA was immediately spin coated onto the sample to protect the flake from being degraded in the air ambient. The source and drain electrodes were precisely patterned on the flake using the conventional e-beam lithography technique, followed by thermal evaporation of Ti (5 nm) and Au (80 nm) as the metal contacts. After liftoff, the as-made devices were wire bonded onto a leaded chip carrier (LCC) and loaded in a custom-designed high vacuum system (~10 −8 mbar) for in situ electrical measurements. In situ device characterization FET characterizations were carried out using an Agilent 2912A source measure unit at room temperature. Cs 2 CO 3 and MoO 3 were separately evaporated in situ from a Knudsen cell onto the devices in high vacuum chamber. The nominal thickness of Cs 2 CO 3 and MoO 3 layers was calibrated by a quartz crystal microbalance exactly located in front of the sample stage. In situ photoresponse measurements were also conducted right after the deposition of doping layers in the high vacuum chamber. The sample was illuminated by a 405-nm laser with power of 40 mW (spot diameter 2.0 mm). In situ UPS and XPS characterization In situ UPS and XPS measurements on both MoO 3 - and Cs 2 CO 3 -coated bulk BP were carried out in a home-made ultrahigh vacuum chamber (10 −10 mbar) with He I (21.2 eV) and Mg Kα (1,253.6 eV) as excitation sources, respectively. By applying a sample bias of −5 V, the sample work function was determined by the secondary electron cutoff at the low kinetic energy region. The nominal thickness of in situ deposited Cs 2 CO 3 and MoO 3 layers was estimated by the attenuation of P 2p 3/2 peak and further calibrated by quartz crystal microbalance. How to cite this article: Xiang, D. et al . Surface transfer doping induced effective modulation on ambipolar characteristics of few-layer black phosphorus. Nat. Commun . 6:6485 doi: 10.1038/ncomms7485 (2015).